Radially aligned hierarchical columnar structure as a cathode material for high energy density sodium-ion batteries Delivery of high capacity with good retention is a challenge in developing cathodes for rechargeable sodium-ion batteries. Here we present a radially aligned hierarchical columnar structure in spherical particles with varied chemical composition from the inner end (Na[Ni 0.75 Co 0.02 Mn 0.23 ]O 2 ) to the outer end (Na[Ni 0.58 Co 0.06 Mn 0.36 ]O 2 ) of the structure. With this cathode material, we show that an electrochemical reaction based on Ni 2+/3+/4+ is readily available to deliver a discharge capacity of 157 mAh (g-oxide) −1 (15 mA g −1 ), a capacity retention of 80% (125 mAh g −1 ) during 300 cycles in combination with a hard carbon anode, and a rate capability of 132.6 mAh g -1 (1,500 mA g -1 , 10 C-rate). The cathode also exhibits good temperature performance even at −20°C. These results originate from rather unique chemistry of the cathode material, which enables the Ni redox reaction and minimizes the surface area contacting corrosive electrolyte. Lithium batteries currently dominate the secondary battery market because of their high energy and good power density. Recently, fossil fuel depletion and air pollution concerns have accelerated the development of mid- and large-scale batteries for vehicles and energy storage devices [1] . The recent launch of several types of electric vehicles powered by rechargeable lithium batteries has necessitated significant improvements in battery performance including higher capacity and power, longer life cycle and improved safety. Despite their feasibility, the mass production of such large-scale batteries would likely contribute to the future exhaustion of limited lithium resources. This concern has led us to look for alternative systems to replace current lithium-related chemistries. Because of sodium’s abundance in nature, sodium-based rechargeable batteries have recently received intensive attentions [2] , [3] , [4] , [5] . Electrochemical insertion/extraction of sodium ion was introduced in the early 1980s (refs 6 , 7 , 8 ) but research has been directed towards lithium systems due to lithium’s higher available energy. Provided that appropriate electrode materials can be discovered, substituting Na for Li should be accelerated due to the similar chemistries between Li and Na systems because Na is substantially less expensive than Li. Recently, several types of insertion materials have been introduced as cathode materials for sodium-ion batteries (SIBs) including P2-types [9] , [10] , [11] , [12] , [13] , [14] , [15] , [16] , O3-types [17] , [18] , [19] , [20] , [21] , [22] , [23] , [24] , [25] , [26] , [27] , [28] , [29] , pyrophosphates [30] , [31] , [32] and organo-compounds [33] , [34] , [35] . Owing to the large ionic size of Na + ions (1.02 Å), their insertion into a spinel framework does not readily occur. In contrast, two-dimensional layer structures do favour the insertion of Na + ions into their structures. Among these, P2- (refs 9 , 10 , 11 , 12 , 13 , 14 , 15 , 16 ) and O3-types [17] , [18] , [19] , [20] , [21] , [22] , [23] , [24] , [25] , [26] , [27] , [28] , [29] , which are classified by their sequence of oxygen stacking, are of interest because of their large reversible capacities. For layer-structured compounds, the P2-type usually stabilizes into Na-deficient compositions such as Na 2/3 MO 2 (M: Ni, Co, Mn, Fe and so on). These compounds exhibit reversible capacity below 150 mAh g −1 . Recently, Komaba et al. [9] suggested a new compound (P2-type Na 2/3 Fe 0.5 Mn 0.5 O 2 ) that delivers 190 mAh g −1 , thereby enabling the use of earth-abundant elements but it shows lower cycle retention of 79% during 30 cycles. O3-type compounds, typically NaMO 2 (M: Ni, Co, Mn, Fe, Cr, V and so on), possess the same crystal structure as LiMO 2 (M: Ni, Co, Mn) [17] , [18] , [19] , [20] , [21] , [22] , [23] , [24] , [25] , [26] , [27] , [28] , [29] . These layer structures are readily synthesized via various methods such as the ceramic method [17] , [18] , [20] , [21] , [25] , [27] , co-precipitation [19] , [22] , [23] , [26] and sol-gel processing [24] . Among them, co-precipitation has been particularly effective for the creation of hydroxide and oxalate structures and can be used to prepare multi-component (Ni-Fe-Mn) hydroxide and oxalate forms that give phase-pure Na[NiFeMn]O 2 products [22] , [23] . A recent study by Mortemard de Boisse et al. [27] demonstrated the better cyclability of O3-type Na x Mn 1/2 Fe 1/2 O 2 relative to P2-type Na x Mn 1/2 Fe 1/2 O 2 (though the initial capacity of the O3-type compound was slightly lower). Also, lower approximate capacities were found for several sodiated layered compounds in O3 type including NaFeO 2 (ref. 18 ), NaNi 0.5 Mn 0.5 O 2 (refs 19 , 26 ), NaFeO 2 -Na[Ni 1/2 Mn 1/2 ]O 2 (ref. 20 ), NaVO 2 (ref. 21 ), Na[Ni 1/3 Fe 1/3 Mn 1/3 ]O 2 (ref. 22 ), Na[Ni 0.25 Fe 0.5 Mn 0.25 ]O 2 (ref. 23 ) and Na[Ni 1/3 Co 1/3 Mn 1/3 ]O 2 (ref. 24 ). To overcome the limited capacity of O3-type cathodes, it is important to create unique morphologies that endow high-capacity, long-term cyclability and high energy density. Through our prior works [36] , [37] , we suggested that the nanorod-structured full concentration gradient materials are beneficial in performing outstanding electrochemical properties and excellent safety in lithium-ion batteries system, because the dense rod assembly could minimize surface area contacting with electrolyte, in which the environment, in turn, renders active materials less exposure in acidic electrolyte due to NaPF 6 salt (HF attack). The aforementioned inspires us that, provided that the rods can be further lengthened with radial distribution the product would have several advantages as follows: (1) reduce the surface area of secondary micron particles by rod-shaped primary particles, (2) increase the Li-ion diffusion rate during charge/discharge along with the direction of nanorod, (3) increase the electrode energy density from the high tap density of micron spherical morphology, (4) increase the discharge capacity through the inner high Ni composition and (5) increase the thermal stability and cycle retention through the outer high Mn composition. In this study, therefore, we propose a highly dense spherical particle composed of a radially assembled columnar structure that hierarchically varies the chemical composition from the inner end, Na[Ni 0.75 Co 0.02 Mn 0.23 ]O 2 , to the outer end, Na[Ni 0.58 Co 0.06 Mn 0.36 ]O 2 , of the spherical particle. The electrochemical activity and structural stability of high-Ni systems have yet to be disclosed in Na systems. Here we report the electrochemical and physiochemical properties of our developed materials using various kinds of method. Radially aligned hierarchical columnar structure We anticipate that the linear variation in the Ni concentration towards the surface of the particle leads to high capacity. To confirm that assumption, we measured the electrochemical performances of Na[Ni 0.60 Co 0.05 Mn 0.35 ]O 2 (bulk), Na[Ni 0.75 Co 0.02 Mn 0.23 ]O 2 (inner) and Na[Ni 0.58 Co 0.06 Mn 0.36 ]O 2 (outer) electrodes. Here we exclude the possibility of electrolytic decomposition, since the employed ethyl methanesulfonate-based electrolyte is stable up to 5.6 V versus Na/Na + as confirmed in the result of linear sweep voltammetry test [23] . As expected, high-Ni-composition materials showed higher discharge capacity than low-Ni-composition materials, similar to layered cathode materials for lithium batteries [38] . Because of the great difference in the ionic radius between Na + (1.02 Å) and Ni 2+ (0.69 Å), incorporation of Ni 2+ into the Na layers or site exchange between Na + and Ni 2+ cations does not likely occur in the crystal structure and does not affect the high-capacity delivery for the high-Ni-composition materials, as priorly reported by several groups [19] , [20] , [23] , [25] , [26] . For example, Li[Ni 0.8 Co 0.1 Mn 0.1 ]O 2 and Li[Ni 0.5 Mn 0.5 ]O 2 have the same theoretical capacity of about 280 mAh g −1 . By contrast, Li[Ni 0.8 Co 0.1 Mn 0.1 ]O 2 (typically 200 mAh g −1 based on Ni 3+/4+ redox in the voltage range of 2.5–4.3 V) delivers much higher capacity than that of Li[Ni 0.5 Mn 0.5 ]O 2 (typically 150 mAh g −1 based on Ni 2+/3+/4+ redox in the voltage range of 2.5–4.3 V). Since the energy level of Ni 3+/4+ redox is lower than that of Ni 2+/3+ , Ni 3+/4+ redox reaction readily occurs relative to that of Ni 2+/3+ , as suggested by Delmas et al. [39] However, the similar capacity of 200 mAh g −1 could be obtained when Li[Ni 0.5 Mn 0.5 ]O 2 was charged to 4.6 V (refs 40 , 41 ). Assuming the theoretical capacity of Li[Ni 0.5 Mn 0.5 ]O 2 to be 280 mAh g −1 that is supported by Ni 2+/3+ of about 140 mAh g −1 and Ni 3+/4+ of about 140 mAh g −1 , one can understand that the delivered capacity of 150 mAh g −1 up to 4.3 V is mainly contributed by the Ni 2+/3+ redox reaction although the related kinetic is slow for the Li[Ni 0.5 Mn 0.5 ]O 2 . From the discussion, it is considered that the related redox species and kinetics would be related to the high-capacity delivery of high-Ni-composition materials. These phenomena are applicable to Na system ( Supplementary Fig. 1 ). Namely, the inner composition, Na[Ni 0.75 Co 0.02 Mn 0.23 ]O 2 supported by Ni 3+/4+ redox provides more capacity than that of outer composition, Na[Ni 0.58 Co 0.06 Mn 0.36 ]O 2 by Ni 2+/3+ to 4.1 V versus Na/Na + though capacity retention is better for the outer composition during cycling. Therefore, hierarchical composition variation was important to achieve both high capacity and stable cycle properties at the same time ( Fig. 1 ). The resulting cycle performance and thermal safety can be compensated by the enrichment of Mn into the outer region. We examined the effect of Mn concentration on the designated radially assembled structure. Supplementary Fig. 2 shows the charge–discharge profiles and cycle performances of these materials for various Mn compositions (0.25<Mn composition<0.35; Ni composition was fixed at 0.6). All of the materials exhibit the same first discharge capacity at 0.1 C-rate because of the same Ni concentration. The cycle retentions of these materials were enhanced with increased Mn composition, which replaced the cobalt in the total composition. From these comparison data, we determined the best composition of our unique radially aligned hierarchical columnar structure (hereafter referred to as RAHC) to be Na[Ni 0.6 Co 0.05 Mn 0.35 ]O 2 for accomplish the superior electrochemical properties. 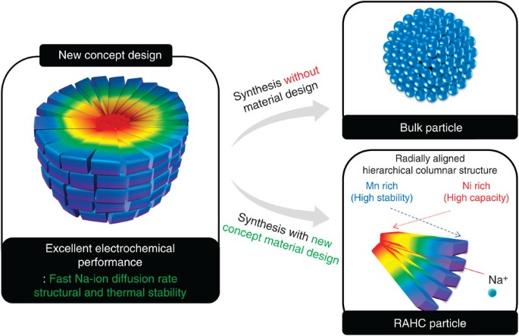Figure 1: Design scheme for a RAHC particle compared with a bulk particle. Left: Representative hemisphere image of new concept design for the cathode materials. Right: (top) Illustration of single particle of conventional bulk cathode materials; (bottom) Illustration of microstructure of radially aligned hierarchical columnar structure of developed cathode materials with new concept design. Figure 1: Design scheme for a RAHC particle compared with a bulk particle. Left: Representative hemisphere image of new concept design for the cathode materials. Right: (top) Illustration of single particle of conventional bulk cathode materials; (bottom) Illustration of microstructure of radially aligned hierarchical columnar structure of developed cathode materials with new concept design. Full size image Advanced structure of high-energy sodium cathode Hydroxides were first synthesized to substantiate the aforementioned concept: hierarchically formed columnar structured spheres in which the chemical composition linearly varies from the inner to outer ends are utilized to form columnar structure ( Fig. 2a ). The resulting X-ray diffraction (XRD) patterns show a typical layer-structure hydroxide: M(OH) 2 (M: metal). The microscopic image of the product indicates a spherical secondary particle with a diameter of ∼ 10 m (inset of Fig. 2a ). Note that the transmission electron microscope (TEM) image clearly demonstrates the radial distribution of the columnar structure from the centre of the particle to the surface, and the columnar structure lengthens to 5–6 μm ( Fig. 2c ). The elemental distribution of the hydroxide was investigated using an integrated two-dimensional electron probe microanalysis; the columnar structure that grew from the centre of the particle to the surface was also analysed ( Fig. 2b ). It is evident that the chemical composition of the hydroxide gradually evolves toward the particle surface: the Ni concentration decreases from 80 to 58 at.%, the Co concentration increases from 2 to 6 at.% and the Mn concentration increases from 18 to 36 at.%. The average chemical composition of the hydroxide was determined to be [Ni 0.60 Co 0.05 Mn 0.35 ](OH) 2 as confirmed by atomic absorption spectroscopy. 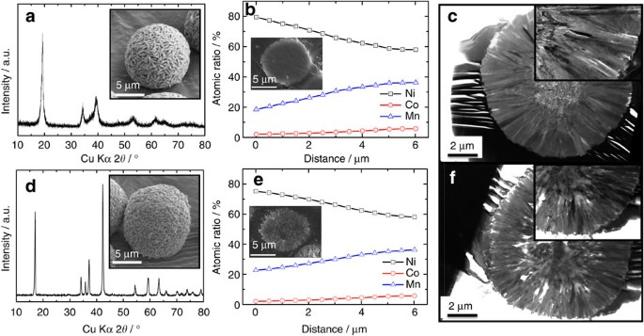Figure 2: Unique concept of RAHC. (a) XRD patterns (inset: scanning electron microscope (SEM) image), (b) Electron probe microanalysis results (inset: cross-sectional SEM image) and (c) cross-sectional TEM image of RAHC [Ni0.60Co0.05Mn0.35](OH)2. (d) XRD patterns (inset: SEM image), (e) EPMA results (inset: cross-sectional SEM image), (f) cross-sectional TEM image of sodiated Na[Ni0.60Co0.05Mn0.35]O2. Figure 2: Unique concept of RAHC. ( a ) XRD patterns (inset: scanning electron microscope (SEM) image), ( b ) Electron probe microanalysis results (inset: cross-sectional SEM image) and ( c ) cross-sectional TEM image of RAHC [Ni 0.60 Co 0.05 Mn 0.35 ](OH) 2 . ( d ) XRD patterns (inset: SEM image), ( e ) EPMA results (inset: cross-sectional SEM image), (f) cross-sectional TEM image of sodiated Na[Ni 0.60 Co 0.05 Mn 0.35 ]O 2 . Full size image Thermal sodiation of the hydroxide at 700 °C results in the formation of an O3-type layer structure belonging to the R-3m space group ( Fig. 2d ). The secondary particle size is not altered after the heat treatment, and shrinkage of the primary particles is likely due to the dehydration of the hydroxide and simultaneous condensation to form an oxide at high temperature (inset of Fig. 2d ). The cross-sectional TEM image of the calcined particle demonstrates that the secondary particle is an assembly of a long columnar structure distributed radially ( Fig. 2f ). We believe that interatomic diffusion of transition metal elements is not likely to occur because the hydroxide morphology was maintained after the heat treatment. Compared with our previous works [42] , this phenomenon could explain through the optimized parameters during synthesis of hydroxide precursor (specifically the optimized amounts of ammonium hydroxide and sodium hydroxide). Through this optimized synthetic method, long rod-shaped primary particles were formed which interrupt the transition metal diffusion because of densely agglomerated morphology. Another clue is the use of NaOH for sodium source. Since the melting point of NaOH is low (318 °C), infiltration of Na element is possible at low temperature that does not influence on interdiffusion of transition metal element during heat treatment. Electron probe microanalysis data confirm the distribution of the transition metal elements along the columnar structure ( Fig. 2e ). These results show that Ni decreases and Co, Mn increases towards the outer end of the columnar structure. This indicates the similarity of the calcined product to the hydroxide in both structure and chemical composition. From the observed diffraction patterns of the sodiated columnar structure (using TEM analysis), we confirmed that the columnar structure showed a layer structure that matched well with our XRD results and the c-axis of the rod-shaped particle was aligned along the tangential direction ( Supplementary Fig. 3 ). The presence of the long columnar structure with a varying chemical composition along its long axis helps to explain the formation of the hierarchically formed columnar structured spheres, as shown in Fig. 1 . Using atomic absorption spectroscopy, the average chemical composition of the product was found to be Na[Ni 0.60 Co 0.05 Mn 0.35 ]O 2 . In addition, the measured tap density was high ( ∼ 2.5 g cm −3 ); this is presumably due to the presence of fewer voids in the columnar structure of the RAHC particle. This high tap density is particularly noteworthy because, to date, there have been no reports in the literature that demonstrate such a high tap density in Ni-rich sodiated cathode materials. Importance of the high tap density of the materials accentuates the resulting volumetric energy density of our RAHC materials ( ∼ 1,177 Wh l −1 ), is greater than other types of microscale-structured cathode materials such as Na[Ni 0.5 Mn 0.5 ]O 2 ( ∼ 1,029 Wh l −1 , Tap density: 2.5 g cm −3 ) [23] , Na[Ni 0.25 Fe 0.5 Mn 0.25 ]O 2 ( ∼ 880 Wh l −1 , Tap density: 2.1 g cm −3 ) [26] , LiFePO 4 ( ∼ 820 Wh l −1 , Tap density: 1.5 g cm −3 ) [43] and LiMn 0.85 Fe 0.15 PO 4 ( ∼ 764 Wh l −1 , Tap density: 1.4 g cm −3 ) [44] . Our novel columnar morphology is considered as a plausible approach to yield high energy density cathode materials for SIBs. Electrochemical performance Before comparing the electrochemical performances of RAHC and bulk materials, we optimized the calcination temperature of each material. As shown in Supplementary Fig. 4 , we selected the optimized materials for electrochemical tests (RAHC: 700 °C, bulk: 680 °C). After optimizing the calcination temperature, we compared the lattice parameters of each material using least-square method ( Supplementary Fig. 4a,d ). Both RAHC and bulk materials have similar lattice parameters, where a =2.9447(3) Å and c =15.7701(2) Å for RAHC, a =2.9445(5) Å and c =15.7698(1) Å for bulk. As-synthesized RAHC and bulk Na[Ni 0.60 Co 0.05 Mn 0.35 ]O 2 were compared with verify the utility of these materials in Na cells ( Fig. 3a,b ). The first charge and discharge curves represent the reversible phase transitions toward the monoclinic P3 phase. These are typically observed in O3-type layer compounds ( Fig. 3a ). [19] , [23] , [24] The delivered discharge capacity reaches ∼ 157 mAh (g-oxide) −1 for the RAHC Na[Ni 0.60 Co 0.05 Mn 0.35 ]O 2 at 15 mA g −1 (0.1 C-rate) and is about 145 mAh (g-oxide) −1 for the bulk material with same composition. The higher discharge capacity of the RAHC would be contributed by two reasons; (1) the directional growth of the primary columnar particles provided extended fast channels for Na + ion diffusion, which was analysed by TEM ( Supplementary Fig. 3 ), (2) the presence of more amount of Ni 3+ along with the long columnar particle towards the centre, which has lower energy level of Ni 3+/4+ than Ni 2+/3+ redox reaction [39] , as seen in the X-ray photoelectron spectroscopy analysis result ( Supplementary Fig. 5 ). From this consideration, although the amount of Ni is same for bulk and RAHC, the obtained capacity of 157 mAh g −1 for the RAHC is the result of not only Ni 2+/3+/4+ but also Ni 3+/4+ redox reactions. For the reason, the capacity of RAHC is higher than that of bulk, though their chemical composition is identical each other. Also, the efficiency is notably high during the first cycle for both electrodes. Half cell cycling tests, measured at 75 mA g −1 (0.5C), indicate that the present RAHC electrode exhibits a highly reversible phase transition and maintains high capacity on cycling at both 30 °C and 55 °C ( Fig. 3b , Supplementary Fig. 6 ). The resulting capacity remains nearly constant at each plateau during cycling, and it still shows high discharge capacity after the 100th cycle (125.7 mAh g −1 at 30 °C, 98.0 mAh g −1 at 55 °C). In contrast, the bulk Na[Ni 0.60 Co 0.05 Mn 0.35 ]O 2 electrode undergoes gradual capacity fading over the entire region. Either the capacity or the retention of the bulk Na[Ni 0.60 Co 0.05 Mn 0.35 ]O 2 is poorer than that of Na[Ni 0.25 Fe 0.5 Mn 0.25 ]O 2 (ref. 23 ) which demonstrates the difficulty of utilizing Ni-rich compounds in Na systems. We also compared the reversibility of the RAHC for bulk electrodes using dQ/dV profiles between the 1st and 100th cycles ( Supplementary Fig. 7 ). Similar to the cycle retention results, the RAHC electrode maintained all of the redox potential peaks clearly after cycling, but the redox peaks of the bulk electrode decreased obviously after 100 cycles. The present concept, which utilizes high-density spherical particles composed of a radially assembled columnar structure that hierarchically varies the chemical composition from the inner end (Na[Ni 0.75 Co 0.02 Mn 0.23 ]O 2 ) to the outer end (Na[Ni 0.58 Co 0.06 Mn 0.36 ]O 2 ) in a spherical particle (RAHC), enables the realization of Ni-based redox reactions that yield high-capacity and stable cycle performance. 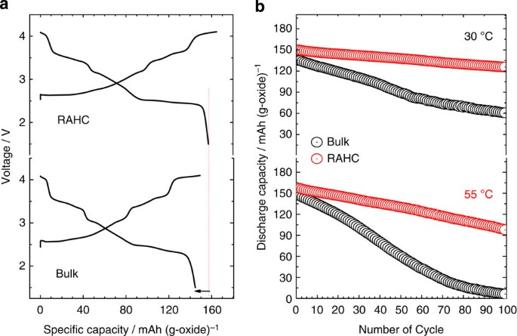Figure 3: Electrochemical characterization. (a) First charge–discharge curves and (b) cycle retention of the RAHC and bulk electrodes using Na metal anode. Figure 3: Electrochemical characterization. ( a ) First charge–discharge curves and ( b ) cycle retention of the RAHC and bulk electrodes using Na metal anode. Full size image Thermal property Thermal stability is another important concern that should be investigated before these electrode materials are deemed suitable for use in alternative power sources. For this reason, powders were chemically or electrochemically desodiated to form Na 0.36 [Ni 0.60 Co 0.05 Mn 0.35 ]O 2 for the RAHC and Na 0.44 [Ni 0.60 Co 0.05 Mn 0.35 ]O 2 for the bulk powders. In these, the extracted amount of Na + ions is equivalent to a charge capacity of 4.1 V, as shown in Fig. 3a,b . Differential scanning calorimetry was used to analyse shifts in the exothermic reactions ( Fig. 4a ). The electrochemically desodiated RAHC Na 0.36 [Ni 0.60 Co 0.05 Mn 0.35 ]O 2 was seen to undergo less heat generation (172 J g −1 at 293.5 °C) at a higher temperature compared with the bulk Na 0.44 [Ni 0.60 Co 0.05 Mn 0.35 ]O 2 (321.6 J g −1 at 266.5 °C). It is worth mentioning that, although a more amount of Na + ions were extracted from the host structure of the RAHC than from the bulk material, the observed reaction appears at a higher temperature with less heat generation. Indeed, the RAHC Na 0.36 [Ni 0.60 Co 0.05 Mn 0.35 ]O 2 should exhibit more heat at lower temperatures compared with the bulk Na 0.44 [Ni 0.60 Co 0.05 Mn 0.35 ]O 2 . Another fact to consider is that the chemical composition of the outer composition is similar for the two samples: Na[Ni 0.58 Co 0.06 Mn 0.36 ]O 2 for the RAHC and Na[Ni 0.60 Co 0.05 Mn 0.35 ]O 2 for the bulk. Therefore, if the surface composition were detrimental to the reaction, both materials would show a similar exothermic reaction. 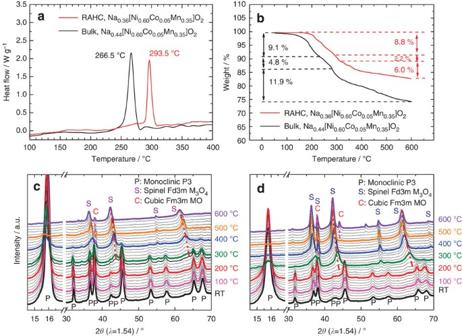Figure 4: Analysis of thermal property. (a) Differential scanning calorimetry results, (b) thermogravimetric analysis results of desodiated RAHC and bulk electrodes andin situhigh-temperature XRD results of (c) RAHC electrode and (d) bulk electrode. Figure 4: Analysis of thermal property. ( a ) Differential scanning calorimetry results, ( b ) thermogravimetric analysis results of desodiated RAHC and bulk electrodes and in situ high-temperature XRD results of ( c ) RAHC electrode and ( d ) bulk electrode. Full size image The thermogravimetric study of the desodiated powders also provided some interesting results. The observed weight loss is nearly identical at the onset temperatures of the exothermic reactions: a weight reduction of 9 wt% occurs for the RAHC Na 0.36 [Ni 0.60 Co 0.05 Mn 0.35 ]O 2 at 290 °C and the bulk Na 0.44 [Ni 0.60 Co 0.05 Mn 0.35 ]O 2 at 240 °C ( Fig. 4b ). This is mainly caused by oxygen release from the crystal structure. The exothermic reaction progresses by releasing more oxygen (4.8 wt% loss) between 240 °C and 280 °C for the bulk Na 0.44 [Ni 0.60 Co 0.05 Mn 0.35 ]O 2 . For the RAHC Na 0.36 [Ni 0.60 Co 0.05 Mn 0.35 ]O 2 , the same exothermic reaction is observed between 280 and 310 °C, but the amount of oxygen that is released is lower (corresponding to a weight loss of 2.2 wt%). The difference in the oxygen content could be related to the degree of heat generated during the exothermic reaction. Even after the exothermic reaction is complete, weight loss varies less for the Na 0.36 [Ni 0.60 Co 0.05 Mn 0.35 ]O 2 up to 600 °C. A high-temperature in situ XRD was employed to observe how the structure of these desodiated powders evolved with increasing temperature ( Fig. 4c,d ). A high-temperature in situ XRD pattern were obtained using a diffractometer at the Center for Energy Convergence Research, Korea Institute of Science and Technology (KIST) and at beamlines 1D and 5A of the Pohang Light Source (PLS, Korea). Both RAHC Na 0.36 [Ni 0.60 Co 0.05 Mn 0.35 ]O 2 and bulk Na 0.44 [Ni 0.60 Co 0.05 Mn 0.35 ]O 2 show a monoclinic P3 phase at room temperature. The structure remains constant up to 260 °C for the RAHC Na 0.36 [Ni 0.60 Co 0.05 Mn 0.35 ]O 2 ( Fig. 4c ), after which a cubic spinel phase is formed at 280 °C (where the exothermic reaction is initiated). Even after the main exothermic reaction at 310 °C, the P3 phase is retained (up to 400 °C); phase transformation to the spinel phase is completed at around 500 °C. A cubic closed-packed MO (M: Ni, Co, Mn) phase is also observed at this point. In contrast, the advent of the spinel phase is observed at 240 °C for the bulk Na 0.44 [Ni 0.60 Co 0.05 Mn 0.35 ]O 2 , and the P3 phase has been drastically transformed to the spinel phase at 280 °C (the point at which the main exothermic reaction occurs). Above 300 °C, the original P3 phase is no longer found in the XRD pattern; the material is dominantly spinel phase with cubic MO (M: Ni, Co, Mn) as a minority. These results demonstrate that the RAHC is thermally stable owing to the slow progress of the phase transformation from monoclinic P3 to cubic MO via an intermediate spinel structure. These phase transformations are driven by oxygen evaporation from the parent crystal structure during heating. Therefore, it appears that the released oxygen content is proportional to the surface area of the primary particles. The measured surface area for the RAHC is about 0.77 m 2 g −1 , whereas the surface area for the bulk material is found to be 6.41 m 2 g −1 ( Supplementary Fig. 8 ). Provided that the involved reaction is initiated from the surface, a smaller surface area would be beneficial for reducing the amount of oxygen removed from the host structure. Indeed, the surface composition is similar for the RAHC and the bulk; therefore, it is expected that the exothermic reaction would occur in a similar method. However, the lower surface area for the RAHC, compared with the bulk, provides less contact with electrolyte in the radially aligned columnar structured spherical particle. This leads to less oxygen being evaporated from the crystal structure. Because the amount of oxygen removed from this structure is less, the phase evolution from monoclinic P3 to the cubic structure is delayed. Therefore, it is possible to understand the better thermal properties of the RAHC from the combined differential scanning calorimetry, thermogravimetric and HT- in situ -XRD studies. It is necessary to investigate the long-term cyclability to confirm the feasibility of the present RAHC cathode. The full SIB used in this work utilizes a hard carbon anode that was presodiated to reduce the irreversible capacity [26] . We used this technique, not for commercial application but, for scientific queries to test long-term electrochemical performance of our materials using full cells, since metallic deposition of Na on the Na metal anode does not warrant long term cycling test. As shown in Supplementary Fig. 9 , presodiated hard carbon electrode shows the reversible discharge capacity of 257 mAh g −1 (Na 0.68 C 6 ) with non-irreversible capacity. From the comparison of the charge–discharge curves of presodiated and as-prepared hard carbon electrodes, we could calculate that the inserted amount of sodium during presodiation is about 0.18 mol per C 6 (Theoretical capacity of hard carbon is about 375 mAh g −1 for NaC 6 ). Although we have suggested carbon-coated Fe 3 O 4 as a promising anode material, we used a hard carbon anode in this study because the conversion electrode lowers the energy density compared to hard carbon due to the higher operation voltage. [23] , [26] Our preliminary data for full cells ( Supplementary Figs 10 and 11 ), both of C/RAHC and C/Bulk full cells, indicate that the optimized condition was to settle the N/P ratio to 1.1 for the full cell fabrication, which was determined based on irreversible capacity and operation voltage varying the ratio from 1.1 to 1.5 ( Supplementary Figs 10a and 11a ). The RAHC Na[Ni 0.60 Co 0.05 Mn 0.35 ]O 2 /hard carbon full cell was tested in the voltage range of 1.5–3.9 V at various temperatures (15 mA g −1 , 0.1 C-rate), as shown in Supplementary Fig. 12 . The delivered capacities of the cell reached 143 mAh g −1 at 30 °C, 147.6 mAh g −1 at 55 °C and 128.8 mAh g −1 at 0 °C. The capacity decreases to 114 mAh g −1 at −20 °C; however, this value is still sufficiently high compared with Li cells [45] , [46] , [47] . At 30 °C, the average operation voltage is found to be 2.84 V on discharge. We tested the 0.5 C-rate long-term cycling of the RAHC/hard carbon full cell during 300 cycles for comparison with the bulk/hard carbon full cell at 30 °C ( Fig. 5a–c ). We additionally measured the pore volume of both materials to analyse these cycle retention results ( Supplementary Fig. 8 ). As expected, the RAHC materials show smaller surface area and pore volume values than the bulk materials do, which means the RAHC materials could avoid the unnecessary reaction with the electrolyte at the surface of the materials. Through these comparison data, we confirmed that the RAHC material shows excellent cycle retention during extensive cycling conditions (RAHC: 80.0%, bulk: 49.2%), which could be achieved via a radially aligned columnar structure that provides small surface area and pore volume. Cycling tests measured at 75 mA g −1 (0.5 C) indicate that the present cathode is suitable for full cell cycling at various temperatures: 83% at 55°C, 89% at 0 °C and 92% at −20 °C during 100 cycles ( Fig. 5d , Supplementary Fig. 13 ). In addition, the rate capability of the RAHC Na[Ni 0.60 Co 0.05 Mn 0.35 ]O 2 /hard carbon full cell is compared with the bulk Na[Ni 0.60 Co 0.05 Mn 0.35 ]O 2 cathode ( Fig. 5e ). The RAHC electrode delivers reversible capacities of ∼ 140.9 mAh g −1 at 1 C-rate, 134.2 mAh g −1 at 5 C-rate and 127.3 mAh g −1 at 10 C-rate, while the discharge capacity is about 81.5 mAh g −1 at 10 C-rate for the bulk Na[Ni 0.60 Co 0.05 Mn 0.35 ]O 2 electrode. We compared electrochemical properties of several O3 and P2 type layered cathode materials to confirm the novelty of the present RAHC material ( Table 1 ). The comparison indicates competitiveness of the RAHC material in terms of capacity, cycle retention even in full cell and high rate capability. The present hierarchical structure from the inner end (Na[Ni 0.75 Co 0.02 Mn 0.23 ]O 2 ) to the outer end (Na[Ni 0.58 Co 0.06 Mn 0.36 ]O 2 ) of the columnar structure assembly is probably responsible for the high-capacity retention during cycling and the good rate performances. These data indicate that the Ni 2+/3+/4+ redox reaction can be utilized to obtain high capacity in O3-type Ni-rich layer compounds, even at high rates, in the RAHC particles. This emphasizes the importance of morphology; using the radial alignment of columnar structure in three-dimensions, enabling reduction of the surface area. Since this morphology minimizes contact with the electrolyte, side reactions are also minimized during long-term electrochemical cycling ( Fig. 5a ). For this reason, the O3-type RAHC is able to retain its high capacity throughout extensive cycling. 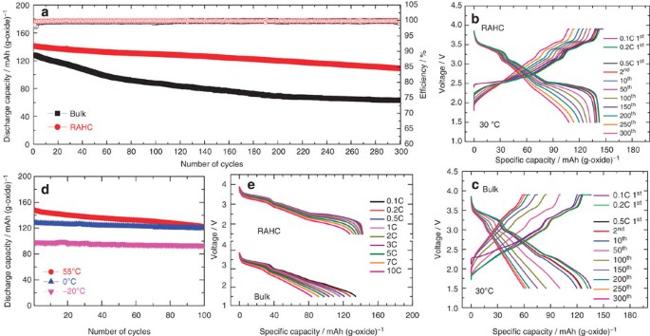Figure 5: Comprehensive overview of electrochemical performance of the C/RAHC and C/Bulk battery. (a) Long-term cycle retention of C/Na[Ni0.60Co0.05Mn0.35]O2RAHC, C/bulk full cells; cutoff: 1.5–3.9 V, current density: 75 mA g−1(0.5 C-rate) and resulting charge–discharge curves for (b) C/RAHC, (c) C/Bulk full cells with formation curves (0.1, 0.2 C-rate); cutoff: 1.5–3.9 V, current density: 15 mA g−1(0.1 C-rate, 1 cycle), 30 mA g−1(0.2 C-rate, 2 cycles) and 75 mA g−1(0.5 C-rate, 300 cycles), (d) cycle retention of C/Na[Ni0.60Co0.05Mn0.35]O2(RAHC) full cells at various operating temperatures (−20 to 55 °C); cutoff: 1.5–3.9 V (kept 3.9 V until 0.1 C for CV), current density: 75 mA g−1(0.5 C-rate) and (e) rate capabilities of C/RAHC and C/bulk full cells; cutoff: 1.5–3.9 V, current density: 15 mA g−1(0.1 C-rate, charge), 15 to 1,500 mA g−1(0.1–10 C-rate, discharge). All cells kept at 3.9 V until 0.02 C-rate (for 0.1 C cycle) or 0.04 C-rate (for 0.2 C cycle) or 0.1 C-rate (for 0.5 C cycle) in the state of charge. Figure 5: Comprehensive overview of electrochemical performance of the C/RAHC and C/Bulk battery. ( a ) Long-term cycle retention of C/Na[Ni 0.60 Co 0.05 Mn 0.35 ]O 2 RAHC, C/bulk full cells; cutoff: 1.5–3.9 V, current density: 75 mA g −1 (0.5 C-rate) and resulting charge–discharge curves for ( b ) C/RAHC, ( c ) C/Bulk full cells with formation curves (0.1, 0.2 C-rate); cutoff: 1.5–3.9 V, current density: 15 mA g −1 (0.1 C-rate, 1 cycle), 30 mA g −1 (0.2 C-rate, 2 cycles) and 75 mA g −1 (0.5 C-rate, 300 cycles), ( d ) cycle retention of C/Na[Ni 0.60 Co 0.05 Mn 0.35 ]O 2 (RAHC) full cells at various operating temperatures (−20 to 55 °C); cutoff: 1.5–3.9 V (kept 3.9 V until 0.1 C for CV), current density: 75 mA g −1 (0.5 C-rate) and ( e ) rate capabilities of C/RAHC and C/bulk full cells; cutoff: 1.5–3.9 V, current density: 15 mA g −1 (0.1 C-rate, charge), 15 to 1,500 mA g −1 (0.1–10 C-rate, discharge). All cells kept at 3.9 V until 0.02 C-rate (for 0.1 C cycle) or 0.04 C-rate (for 0.2 C cycle) or 0.1 C-rate (for 0.5 C cycle) in the state of charge. Full size image Table 1 Comparison of electrochemical properties of various cathode materials. Full size table In summary, the hierarchically formed columnar structured spheres show that an O3-type layer compound can deliver high capacity, good retention and rate capability and thermal stability at the same time. And these excellent properties were not ever achieved in previous sodium related papers. In particular, the high capacity derived from the Ni 2+/3+/4+ redox reaction is remarkable in a Na system that delivers high capacity. In addition, the smaller surface area provided by the radially aligned long columnar structure is beneficial for reducing the contact area with the electrolyte. This results in less electrochemical and thermal decomposition of the active material. Through further optimization of the electrolyte and the anode, we believe that the suggested RAHC can be used as the cathode material for rechargeable sodium batteries. These batteries should be able to compete with lithium batteries in terms of cost, battery performance and safety. Synthesis of RAHC materials Spherical particles, made up of [Ni 0.6 Co 0.05 Mn 0.35 ](OH) 2 assembled with a radially aligned columnar structure on which the chemical composition hierarchically varies from the inner end to the outer end, were synthesized via co-precipitation [36] , [37] . Two solution tanks were used to control the concentrations of the transition metals. To produce a hierarchical columnar structure, an Ni-poor aqueous solution (tank 2, molar ratio of Ni:Co:Mn=0.58:0.06:0.36) consisting of NiSO 4 ·6H 2 O, CoSO 4 ·7H 2 O and MnSO 4 ·5H 2 O was slowly pumped from tank 2 into an Ni-rich (molar ratio of Ni:Co:Mn=0.80:0.02:0.18) stock solution (in tank 1). The homogeneously mixed solution in tank 1 was then fed into a continuously stirred tank reactor (4L) in a replenished N 2 atmosphere. After the composition of tank 1 reached the desired surface composition, feeding from tank 2 was stopped. Concurrently, a 4.0-mol l −1 NaOH solution (aq.) and the desired amount of a NH 4 OH chelating agent solution (aq.) were separately pumped into the reactor. The concentration of the solution (2 mol l −1 for metal solution), pH (11), temperature (50 °C) and stirring speed of the mixture in the reactor (1,000 r.p.m.) were carefully controlled. During the initial stage of the co-precipitation process, [Ni 0.80 Co 0.02 Mn 0.18 ](OH) 2 (the centre composition) was precipitated first. Nickel-cobalt-manganese hydroxide with a different composition gradually covered the [Ni 0.80 Co 0.02 Mn 0.18 ](OH) 2 particles, resulting in a linear composition change in Ni, Co and Mn towards the outer end (surface) of the particles. The precursor powders were obtained by filtering, washing and drying at 100 °C overnight. The obtained spherical hydroxide, assembled with radially aligned hierarchical columnar structures of varying chemical composition, was thoroughly mixed with NaOH, and the mixture was calcined at 700 °C for 24 h in air. Additional methods details appear in the Supplementary Information . How to cite this article: Hwang, J.-Y. et al. Radially aligned hierarchical columnar structure as a cathode material for high energy density sodium-ion batteries. Nat. Commun. 6:6865 doi: 10.1038/ncomms7865 (2015).